Measuring the size of individual particles from three-dimensional imaging experiments Often experimentalists study particulate samples that are nominally monodisperse. In reality, many samples have a polydispersity of 4–10%. At the level of an individual particle, the consequences of this polydispersity are unknown as it is difficult to measure an individual particle size from images of a dense sample. Here we propose a method to estimate individual particle radii from three-dimensional data of the particle positions. We first validate our method with simulations. We then apply our method to experimental data of colloidal suspensions observed with confocal microscopy. We demonstrate that we can recover the full particle size distribution in situ . Finally, we use our method to study the relationship between homogeneous colloidal crystal nucleation and particle sizes. We show that nucleation occurs in regions that are more monodisperse than average. A wide variety of techniques exist for three-dimensional (3D) imaging of collections of particles, such as granular materials, soils and colloidal suspensions [1] , [2] . Our particular interest is in colloidal suspensions; these have been successfully used as model systems for understanding phase transitions for several decades [3] , [4] , and are interesting in their own right owing to industrial relevance [5] . Confocal microscopy can be used to take 3D images of fluorescent colloidal particles deep within a sample [2] , [6] , [7] . When coupled with particle tracking techniques, the motion of thousands of individual colloidal particles can be followed over long periods of time [8] , [9] , [10] . This technique has been used to investigate the colloidal glass transition [7] , [8] , [9] , [11] , crystallization [12] , [13] , [14] , colloidal gels [15] , [16] , [17] , capillary waves [18] , [19] , sedimentation [12] , [20] and a variety of other questions (see ref. 2 for a review). One advantage of confocal microscopy of colloids is that particle tracking data are similar to simulations that also provide particle positions over long periods of time. However, experimental samples are always polydisperse: even for a nominally single-component sample, the particles have a variety of sizes [21] . This is quantified by the polydispersity p , defined as the s.d. of particle radii divided by the mean radius. For many samples, p ∼ 0.04–0.10 (ref. 21 ). Numerical simulations show that the effects of the particle size distribution are not negligible. For example, crystal nucleation is difficult or impossible for more polydisperse samples [22] , [23] . The crystal–liquid phase boundary depends on the polydispersity [24] . The sensitivity to volume fraction near the glass transition depends on the composition in nontrivial ways [25] , [26] . Experimentally, the influence of polydispersity on colloidal crystallization has been demonstrated [27] , [28] , and there is also some understanding of how polydispersity influences the rheological behaviour of a colloidal sample [29] . However, these are limited to studies of the spatially averaged properties of the sample. Microscopy is useful for local properties, but particle size fluctuations of a few per cent are not easily detectable. It would be desirable to know particle sizes for more direct comparison with simulations. Furthermore, in some cases, neglecting these sizes in an experiment can lead to wrong conclusions. One example is that the pair correlation function g ( r ) can show a qualitatively incorrect dependence on control parameters if the particle sizes are treated as all identical [30] . A second example is that the apparent compressibility of a random close-packed sample depends qualitatively on whether individual particle sizes are taken into account [31] , [32] , [33] . In this work, we introduce a general method for using 3D data to determine the size of individual particles in any moderately concentrated sample, in general with volume fractions φ ≳ 0.4. We use simulation data to verify that our method works well in a variety of sample types. We then check our method with experimental data from confocal microscopy, which compares well with data on the same samples from holographic microscopy. Finally, we demonstrate the utility of our method using previously published experimental data from confocal microscopy of colloids. In particular, we show that colloidal crystal nucleation is sensitive to the local polydispersity: nucleation happens in locally monodisperse regions. Our method is not limited to confocal microscopy and colloidal samples, but rather works with any data of the 3D positions of a collection of particles. Size estimation algorithm Owing to diffraction limits, it is difficult to directly determine the radii of individual particles from microscopy images to better than ±0.1 μm (ref. 34 ). Defining the edge is somewhat arbitrary and varies depending on particle properties and the details of the illumination. Other 3D imaging techniques have similar issues [1] . In contrast, it is much easier to calculate the mean radius ā of particles with a variety of techniques [21] . Likewise, from the centres of particles, the separations between neighbouring particles r ij can be easily calculated. Our estimation method for particle sizes uses only ā and r ij . The key idea of our method is that a large particle will be slightly farther from its neighbours and thus have larger values for its r ij , and likewise a smaller particle will have smaller values of r ij . To start, we relate the pairwise separations r ij as where particle j is a nearest neighbour particle of particle i , r ij is the measured distance between i and j , a i and a j are their radii, and δ ij ( t ) is a surface-to-surface distance between their particles. These distances are sketched in Fig. 1a . When choosing neighbours, we use the particles j that are closest to i (smallest separations r ij ). Typically, we use Z =5–7 of these closest neighbour particles; this choice is justified below. Often these data come from particle tracking, and so r ij ( t ) and δ ij ( t ) depend on time t . Next, we take an average of r ij with respect to the nearest neighbour particles j , and then 〈 r ij ( t )〉 j = a i +〈 a j 〉 j +〈δ ij ( t )〉 j , where 〈〉 j means an average over particle j . 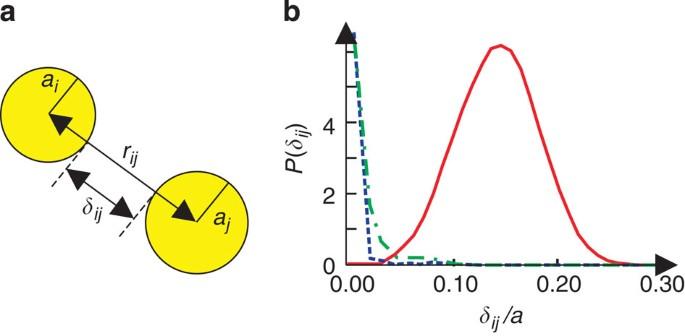Figure 1: Probability distribution function ofδij. (a) Sketch defining key distances. (b) Probability distribution function ofδijfrom simulation data for several systems. The systems and the number of neighboursZin each case are: a dense liquid withφ=0.51 (solid red curve,Z=7), a random close-packed sample (dashed blue curve,Z=5) and a colloidal gel (dash-dotted green curve,Zi=5ci/13). The details of the choices ofZare discussed in the text. Thus, we obtain Figure 1: Probability distribution function of δ ij . ( a ) Sketch defining key distances. ( b ) Probability distribution function of δ ij from simulation data for several systems. The systems and the number of neighbours Z in each case are: a dense liquid with φ =0.51 (solid red curve, Z =7), a random close-packed sample (dashed blue curve, Z =5) and a colloidal gel (dash-dotted green curve, Z i =5 c i /13). The details of the choices of Z are discussed in the text. Full size image This is exact, but the quantities δ ij ( t ) are unknown. We estimate this by replacing δ ij ( t ) with its time- and particle-averaged value, the mean gap distance , where the average is over all particle pairs and all times. Our algorithm is then: where the superscripts denote iteration. The more we iterate equation 4, the more information we obtain from particles far away from a given particle. In fact, is unchanged for n ≥10 as includes the information from several thousand particles, thus we fix n =10 for the number of iterations in this paper. Of course, the particle radius does not depend on time, so after the 10th iteration, we time average ( t ) to obtain the estimated particle radius . Time averaging after each iteration of equation 4 does not change the results. Uncertainty of the estimation There are several sources of uncertainty in this estimation. First, there is the uncertainty of each particle position. Typically this is about 5–8% of the mean radius, leading to a 8–10% uncertainty of r ij (refs 10 , 35 ). However, these errors are nearly time-independent, so those errors are greatly diminished by time averaging. Second, our approximation for δ̄ is weaker in the case that the distribution of δ ij ( t ) is broad. Distributions of δ ij are shown in Fig. 1b . As we choose neighbouring particles j to be those closest to particle i , choosing more neighbours results in a broader distribution of δ ij because the additional neighbours have a larger δ ij by construction. That is, δ̄ increases monotonically with increasing Z . However, using too few neighbours means that the average 〈 r ij ( t )〉 in equation 4 is poor. Below, we use simulation data to determine that Z =5–7 nearest neighbours is an optimal choice. Third, independent of a given choice of Z , some particles will simply be farther from their neighbours, and some will be closer. For example, in a dense suspension this relates to the size of the 'cage' formed by the nearest neighbour particles [9] . Again, time averaging helps. If particles can rearrange and find new neighbours, then δ̄ becomes a better approximation for 〈δ ij ( t )〉 t . Fourth, an additional approximation is that we use to go from equation 2 to equation 4, which assumes that δ ij is uncorrelated with the particle size a i . Our simulations suggest that this is reasonable, but one can imagine situations where it might not be (for example, with charged particles where the charge depended on particle size). In summary, the greatest strength of our algorithm is time averaging, and past that, a sensible choice for the number of nearest neighbours Z is useful. Our tests show that time averaging over ∼ 20 different times is sufficient for reasonable results. Verification of the estimation To verify our radius estimation method, we simulate a variety of systems and compare the estimated radius of each particle with its true radius. The error is given by , where is the estimated value and a i is the true value. is the mean fractional error in the estimated particle radius. Also relevant is the polydispersity p of the simulated sample, defined as , where the averages are over all particles i . A priori , the best guess for each particle size is ā with a fractional uncertainty p . If the mean estimation error Δ a is less than p , the estimation method improves our knowledge of the particle sizes; we will show this is true for the simulated data. Our first test case is a random close-packed sample. In such a sample particles do not move, and so time averaging cannot be used. However, particles are packed so that they can contact each other, that is, δ̄ is close to zero. The number of contacting neighbours varies from particle to particle, so it is not clear how many neighbours should be considered. Accordingly, we plot Δ a as a function of Z in Fig. 2a . We find that Δ a is a minimum at Z =5, and is much smaller than p (0.01 versus 0.07 in this case). In practice we find that the Z =5 closest neighbours are nearly always in contact, and δ̄ ≈ 10 −4 a . 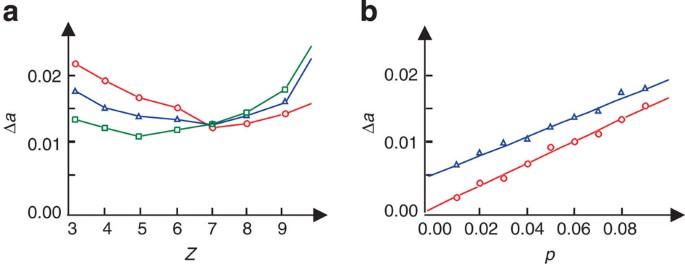Figure 2: Dependence of estimation uncertainty Δaon parameters. (a) The uncertainty Δaas a function of the chosen number of neighboursZused for the averaging. The circles, triangles and squares correspond to Δafor volume fractionsφ=0.51, 0.56 and 0.64 (RCP), respectively. In each case, the sample polydispersity isp=0.07. (b) Δaas a function of the bulk polydispersityp. The circles and the triangles correspond to Δaat RCP andφ=0.51, respectively. The solid lines are the fitting lines for Δa. Figure 2a shows that increasing Z to include some non-contacting neighbours only increases the uncertainty a small amount. Figure 2: Dependence of estimation uncertainty Δ a on parameters. ( a ) The uncertainty Δ a as a function of the chosen number of neighbours Z used for the averaging. The circles, triangles and squares correspond to Δ a for volume fractions φ =0.51, 0.56 and 0.64 (RCP), respectively. In each case, the sample polydispersity is p =0.07. ( b ) Δ a as a function of the bulk polydispersity p . The circles and the triangles correspond to Δ a at RCP and φ =0.51, respectively. The solid lines are the fitting lines for Δ a . Full size image It is possible that while Δ a is small, that there are systematic errors depending on the real particle size a i . To test this, in Fig. 3a we show the ratio between the estimated radius and the given radius as a function of a i for a polydispersity p =0.07 random close packing (RCP) sample. The symbols and the error bars correspond to the mean and s.d. of the distribution of between [ a i , a i +0.01], respectively. should be 1 if our estimation is perfect and indeed we find . The quality of the results is nearly uniform as a function of particle size. To check the validity of our method for RCP samples with different polydispersity, we plot the uncertainty Δ a as a function of sample polydispersity p in Fig. 2b . We find Δ a ≈ p /6 (ref. 33 ). 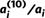Figure 3: The estimated radiusas a function of the true radiusaifor four simulated systems. (a) RCP, (b) a colloidal gel atφ=0.10, (c) a nominally monodisperse suspension atφ=0.51 and (d) a nominally binary suspension atφ=0.51. For (a–c), the polydispersities arep=0.07. For the binary sample, the size ratio is 1:1.3, the number ratio is 1:1, and each species has an individual polydispersity ofp=0.04. The error bars correspond to the s.d. of ofbetweenaiandai+0.01. The insets show sketches of each system. Figure 3: The estimated radius as a function of the true radius a i for four simulated systems. ( a ) RCP, ( b ) a colloidal gel at φ =0.10, ( c ) a nominally monodisperse suspension at φ =0.51 and ( d ) a nominally binary suspension at φ =0.51. For ( a – c ), the polydispersities are p =0.07. For the binary sample, the size ratio is 1:1.3, the number ratio is 1:1, and each species has an individual polydispersity of p =0.04. The error bars correspond to the s.d. of of between a i and a i +0.01. The insets show sketches of each system. Full size image A colloidal gel shares a similarity to a RCP sample (touching or nearly touching particles), and has a significant difference (much lower volume fraction). As an example of how to adapt our algorithm, we consider a simulated depletion gel [36] . In a colloidal gel, particles are stuck to their neighbours and form a large network. Often the attractive interactions have a range, which is true for depletion gels (see discussion in Methods). Thus the distribution of δ ij for gels can be slightly broader than that for RCP, as shown in Fig. 1b , though the mean average of δ ij is close to 0. Some time averaging is possible, although such samples are frequently nonergodic. The contacting particles make gels similar to RCP samples locally. However, the contact number can fluctuate greatly in a colloidal gel. Therefore, rather than fixing the number of neighbours Z to average over, we use Z i neighbours for the average (equation 4). To determine Z i , we define the coordination number c i as the number of particles within a distance 2.8 a of particle i , where 2.8 a is the first minimum of the pair correlation function. We find the average coordination number for a RCP sample, but this can be smaller for some gels [15] . Thus for every particle we select the number of neighbours using Z i =5 c i /13 where we round Z i to the nearest integer, and as always we select the Z i particles closest to particle i to be the neighbours. For tenous gels at dilute concentrations, for many particles Z i is fairly small; also, δ ij has a broader distribution, and so Δ a will be worse than the RCP case. However, Δ a is improved by time averaging. Figure 3b shows the ratio between the time-averaged estimated radius and the given radius as a function of the true radius a i for the colloidal gel. We find that . Δ a =0.018 is much smaller than the polydispersity p =0.070. Moving from gels, we next consider a dense suspension of purely repulsive (hard-sphere) particles. Here, no particles are in contact, so δ ij has a much broader distribution ( Fig. 1b ); however, time averaging is even more powerful. We show as a function of a i at φ =0.51 in Fig. 3c , finding . Yet again Δ a =0.014 is much smaller than the polydispersity p =0.070. For a dense suspension, it is not obvious how many nearest neighbours should be used in the average (equation 4), so we plot Δ a as a function of Z in Fig. 2a for two different volume fractions. Δ a is minimized at Z =7 for the non-RCP samples (circles and triangles in the figure), so we fix our choice Z =7 for all our φ<0.6 experimental data (discussed below). Figure 2a demonstrates that Δ a does not depend too sensitively on this choice. However, it should be expected that for a more dilute system, the importance of caging decreases, and the number of neighbours a particle has will fluctuate significantly. For fixed polydispersity p =0.070, we find Δ a =0.023 for φ =0.45 and Δ a =0.060 for φ =0.40. This suggests that for φ ≲ 0.40, the estimation method may not be useful without further modifications. To check the influence of the sample polydispersity at fixed φ =0.51, we vary p with results shown in Fig. 2b (triangles). We find Δ a ≈0.005+ p /7, suggesting that the estimation is useful for samples with p >0.01, that is, any realistic sample. Δ a is non-zero when p =0, in contrast to the RCP case. This is due to the distribution of δ ij in a dense but non-contacting sample. The last case we examine with simulation data is a nominally binary sample. We simulate a dense suspension composed of particles with a size ratio 1:1.3 (mean sizes 0.877 and 1.14) and number ratio 1:1. For both 'small' and 'large' particles, there is a polydispersity p =0.04. The results are shown in Fig. 3d, and we find at φ =0.51. (Here we have fixed Z =7.) Again, there is no strong dependence on the true particle size a i . However, the uncertainty Δ a for the binary mixture is larger than what is found for the nominally monodisperse distribution. This is consistent with the overall polydispersity of the sample being larger, p =0.14. An important use of our technique is to measure a particle size distribution in situ ; we wish to validate this idea with the simulation data. To do this, we compare the estimated radius distribution with the true radius distribution P ( a i ) in Fig. 4a,b . In both the nominally monodisperse sample and the nominally binary sample, the estimated distribution (symbols) is quite close to the true distribution (curves). We find that for a single-species sample with a Gaussian distribution of radii with polydispersity p , the apparent polydispersity is . Given that for most situations we have shown , our technique will only slightly increase the apparent polydispersity of a sample. 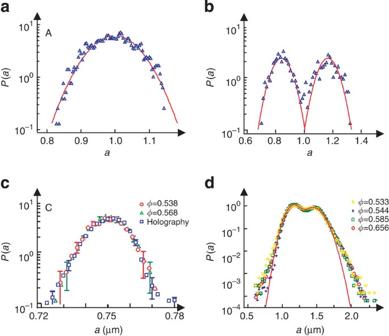Figure 4: Particle size distributions. (a) The distribution of the true radius (solid curve) and the estimated radius(triangles) for a simulated nominally monodisperse sample withφ=0.51 and polydispersityp=0.07. (b) The distribution of the true radius (solid curve) and the estimated radius(triangles) for a simulated nominally binary sample withφ=0.51; see text for more details. (c) The radii distributions for a nominally monodisperse experimental suspension, for two volume fractions as indicated. The blue square symbols are a separate determination of the particle size distribution from holographic microscopy. Representative error bars are shown forP(a); see text for discussion. (d) The radii distributions for the nominally binary experimental suspension from ref.11, for four volume fractions as indicated. Here, the solid curve is a fit to the sum of two Gaussians. With the size ratio (1:1.3) and the polydispersity of each species (p=0.049 for the small species andp=0.050 for the large species), the two subdistributions have substantial overlap. Figure 4: Particle size distributions. ( a ) The distribution of the true radius (solid curve) and the estimated radius (triangles) for a simulated nominally monodisperse sample with φ =0.51 and polydispersity p =0.07. ( b ) The distribution of the true radius (solid curve) and the estimated radius (triangles) for a simulated nominally binary sample with φ =0.51; see text for more details. ( c ) The radii distributions for a nominally monodisperse experimental suspension, for two volume fractions as indicated. The blue square symbols are a separate determination of the particle size distribution from holographic microscopy. Representative error bars are shown for P ( a ); see text for discussion. ( d ) The radii distributions for the nominally binary experimental suspension from ref. 11 , for four volume fractions as indicated. Here, the solid curve is a fit to the sum of two Gaussians. With the size ratio (1:1.3) and the polydispersity of each species ( p =0.049 for the small species and p =0.050 for the large species), the two subdistributions have substantial overlap. Full size image One key difference between simulations and experiments is the boundary condition. Our simulations have periodic boundaries. In an experiment, we cannot find all nearest neighbours of a particle when the particle is located at the edges of an image. This situation is similar to colloidal gels, where the number of nearest neighbours varies for each particle, and we adopt the same solution used there. For each particle, we average over a number of nearest neighbours given by Z i =7 c i /13, where c i is the observed coordination number defined before, and we round Z i to the nearest integer. The denominator 13 is chosen as the number of neighbours in a close-packed sample, and the numerator 7 is from the results of Fig. 2a . Furthermore, we need one more improvement when we apply our method to a nominally binary sample. It usually happens that we know the mean radii a 1 and a 2 of the two subspecies, while the number ratio of two species is unknown, which means that ā is unknown. In this situation, we start with a reasonable guess for ā ′ to be used in equation 3. Then we compute the particle radii and obtain the double peak distribution, which depends on our guess ā ′. The two peaks of the distribution will be at radii a 1 and a 2 : these will differ from the true values. However, the difference will be the same for both, that is, . Adding this difference onto all of the data corrects the distributions and also identifies the true ā . Application to experimental data We now apply our method to experimental data taken on fluorescent silica particles. The particles have a mean radius a =0.752 μm and polydispersity p =0.015, both determined by holographic microscopy [37] , [38] . Holographic microscopy is a powerful technique, which can measure individual particle sizes to high accuracy (uncertainty Δ a / a ≲ 0.005). Using techniques similar to ref. 38 , we determine the sizes of more than 8,000 particles, (see Methods). From these images, we determine the radius of each particle, and show the distribution of radii in Fig. 4c (blue squares). We additionally take 3D confocal microscopy movies of two high-volume fraction samples composed of the same silica particles and apply our method to determine the particle sizes from more than 4,000 particles per sample. These results are plotted in Fig. 4c (circles and triangles). To estimate the uncertainty of P ( a ), we take our list of a data and add additional Gaussian-distributed random noise to each value, with width corresponding to the uncertainty of a based on the technique (holography or our estimation technique). We then compute the new P ( a ): repeating this process 10,000 times gives us fluctuations for P ( a ) for each value of a , shown in the error bars for the three distributions plotted in Fig. 4c . The quantitative agreement between these results is strong evidence that our method works. Note that holographic microscopy works best with dilute samples, whereas our analysis works best with dense suspensions. Separate evidence that our method works is shown in Fig. 4d . Here, we analyse previously published experimental data from ref. 11 (a nominally binary sample, composed of poly-methyl-methacrylate particles). Data from several different volume fractions are shown. Each different volume fraction was a sample taken from the same stock jar and therefore should have the same size distribution, as we observe, confirming the results are robust over a range of volume fractions. A strength of our algorithm is that it only depends on data from the centres of particles. It therefore will work well with core-shell particles (dyed cores and transparent shells), for which the full size of the particle is not optically apparent. It would also work with particles with inhomogeneous dye distributions, so long as their centres could be identified. However, one limitation is that homogeneously dyed particles that are close together have overlapping images that pulls their apparent centres closer together [39] . This may somewhat average out for a random close-packed sample (with neighbours on all sides), but for a gel sample it would be more problematic. Measures can be taken to avoid such errors [39] , [40] , [41] , and using core-shell particles minimizes the problems. In addition, time averaging allows particles to explore different environments and these errors should cancel out over time for samples other than gels and close-packed samples. A second limitation is that systematic and correlated errors can exist in the particle positions. For example, if the calibration (microns/pixel) is slightly incorrect for the z axis, then particles separated in z will have systematic errors in their separation. To mimic an incorrect z calibration, we reconsider the p =0.06, φ =0.51 data and multiply all the z coordinates of the simulation data by 0.98 before we do the radius-estimation algorithm. We find that Δ a only slightly increases (from 0.013 to 0.015). An additional concern is that owing to optical limitations, particle positions are inherently more uncertain in z than in x and y (refs 2 , 6 , 7 , 10 ). For time averaging to be helpful in solving these systematic problem, it would require particles to rearrange significantly during the observation period. Such time averaging is impossible or difficult for random close-packed samples, gels and glassy samples, and so such samples would be more prone to these types of systematic errors. On the other hand, having neighbours distributed in a spherically symmetric fashion around the central particle will help average out the errors to some extent. A third limitation is that charged particles with a polydispersity of charge would have their apparent radii influenced by both their core size and their charge. Probably their estimated radii would depend on a combination of these effects. For example, the estimated radius might relate to the distance where the pairwise particle interaction energy is of magnitude k B T (ref. 42 ). We now demonstrate the utility of our algorithm by studying colloidal crystal nucleation. The nucleation of crystals in a dense particle suspension depends sensitively on polydispersity [23] , [27] , [28] . We examine data of the φ =0.46 sample from ref. 9 , analysed at longer times to examine the crystallization process that was discarded from the analysis in ref. 9 . These particles are slightly charged, shifting the freezing point to φ f reeze ≈0.38 and the melting point to φ m elt ≈0.42 (ref. 13 ). In this data, we confirm that the crystal nucleus appears at the centre of our microscopic image: this is homogeneous nucleation, not heterogeneous nucleation near the wall. At each time step, we calculate the number of ordered neighbours N o for each particle using standard techniques [13] , [43] (see Methods). By convention, a crystalline particle has N o ≥8. At each time, we compute the number fraction of the sample that is crystallized, X ( t ). 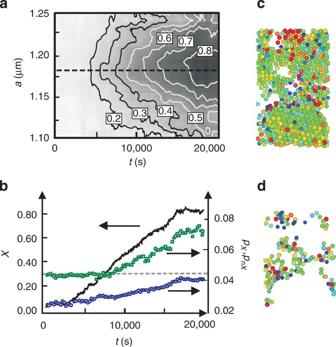Figure 5: Relationship between individual particle sizeaiand crystallization. (a) The contour plot of the fraction of crystalline particlesXas a function ofaiand timet. The contour lines are numbered by the value ofX. The dashed line shows the mean radiusā. Particles with radii close toācrystallize faster. (b) The fraction of the sampleXthat is crystalline as a function of time (solid black curve), along with the mean polydispersity of all crystalline particles (blue circles) and all non-crystalline particles (green squares). The grey dashed line corresponds to the bulk polydispersityp=0.045. (c) The crystalline particles are shown att=20,000 s. (d) The non-crystalline particles are shown att=20,000 s. For (c,d), the colour indicatesaifor each particle, where blue corresponds to smallerai, light green corresponds toaiclose toāand red corresponds to largerai. Figure 5a shows X ( t ) as a function of both individual particle size and time, where darker colours correspond to larger values of X ( t ). Below t =3,000 s, X <0.2 for all a , and essentially all crystal clusters are below the critical size ( ∼ 100 particles) [13] . At t =3,000 s, a sufficiently large crystalline region appears and begins to grow. X increases first for particles with a close to the mean radius, and these particles continue to be the subpopulation that is the most crystallized at any given time. At longer times, the particles with a farther from ā gradually begin to crystallize. Figure 5: Relationship between individual particle size a i and crystallization. ( a ) The contour plot of the fraction of crystalline particles X as a function of a i and time t . The contour lines are numbered by the value of X . The dashed line shows the mean radius ā . Particles with radii close to ā crystallize faster. ( b ) The fraction of the sample X that is crystalline as a function of time (solid black curve), along with the mean polydispersity of all crystalline particles (blue circles) and all non-crystalline particles (green squares). The grey dashed line corresponds to the bulk polydispersity p =0.045. ( c ) The crystalline particles are shown at t =20,000 s. ( d ) The non-crystalline particles are shown at t =20,000 s. For ( c , d ), the colour indicates a i for each particle, where blue corresponds to smaller a i , light green corresponds to a i close to ā and red corresponds to larger a i . Full size image We next consider an alternate way of thinking about the same data. Figure 5b shows the relationship between the sample-averaged X ( t ) (solid black curve), the polydispersity p X for all crystalline particles (blue circles), and the polydispersity p nX for all non-crystalline particles (green squares). X starts to increase at t =3,000 s, and those particles that are crystalline at that time have p X ∼ 0.03, smaller than the bulk polydispersity p =0.045. As the sample crystallizes, we observe that both p X and p nX increase. The growth of p X indicates that the crystal, while nucleating in a fairly monodisperse region, can grow by incorporating particles that are farther from the mean size. In the final state, the local polydispersity of the crystalline particles has nearly reached the mean polydispersity p . The growth of p nX indicates that those particles that are still outside the crystal are more likely to be those with unusual sizes. The spatial distribution of particles at the end of the experiment is shown in Fig. 5c,d . Figure 5c shows the locations of the crystalline particles, while D shows the locations of the non-crystalline particles. Green particles have a i close to ā , and preferentially occupy the cores of the crystal regions. Next, we examine the beginning of the crystal nucleation process. While many particles are close to the mean size, only a few end up being the nucleation site. To understand which ones nucleate, we now focus on the particles close to the mean size: radii 1.175 μm < a i <1.185 μm. Among those particles, we define the nucleus particles as those that are crystalline particles at t =5,000 s, the remainder are non-nucleus particles. We next define the local polydispersity p i ( r ) of particle i as where the angle brackets 〈〉 indicate an average over all particles j with centres within a distance r from particle i . 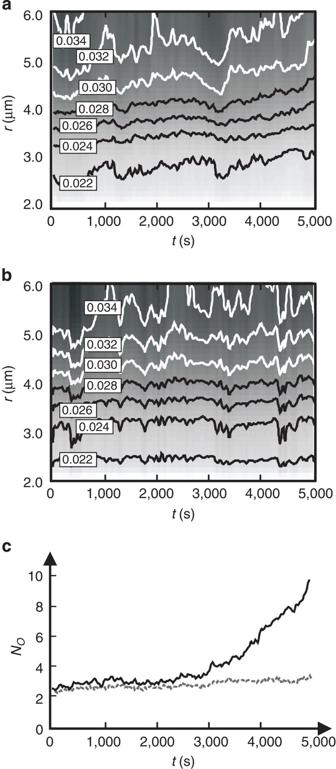Figure 6: Relationship between nucleation properties and the local polydispersitypi(r). (a) The contour plot of the meanpi(r) as a function ofrandt, averaged over all particles that are crystalline att=5,000 s. The numbers on the contour lines represent the value ofpi(r). (b) The contour plot of the meanpi(r) as a function ofrandt, averaged over all particles that are non-crystalline att=5,000 s. The particles considered in (a) and (b) are only those with radii close to the mean radii; see text for details. (c) The number of ordered neighboursNoas a function of time for those particles plotted in (a) (nucleus particles, solid curve) and (b) (non-nucleus particles, dashed curve). Figure 6a,b show space-time plots of the mean value of p i ( r ) for the nucleus particles ( Fig. 6a ) and the non-nucleus particles ( Fig. 6b ). In all cases, p i ( r ) is lower close to the particles and increases with increasing r . However, notably the contours for low p i are at larger values of r for the nucleus particles ( Fig. 6a ): the region of low polydispersity is larger for these particles. After t ≈3,000 s, the region of low p i slightly spreads to even larger values of r for the nucleus particles ( Fig. 6a ), while little change is seen for the non-nucleus particles ( Fig. 6b ). Simultaneously, we show the temporal change of N o in Fig. 6c for the nucleus particles (solid black curve) and the non-nucleus particles (dashed grey curve). This confirms that the onset of crystallization at t ≈3,000 s coincides with the expansion of the low local polydispersity region seen in Fig. 6a . This is all evidence that crystal nuclei are formed from regions where the particles are all similar sizes. A conjecture is that nucleation rates are possibly sensitive to how well mixed the sample initially is: poorly mixed samples with regions of lower local polydispersity will crystallize faster. Figure 6: Relationship between nucleation properties and the local polydispersity p i ( r ). ( a ) The contour plot of the mean p i ( r ) as a function of r and t , averaged over all particles that are crystalline at t =5,000 s. The numbers on the contour lines represent the value of p i ( r ). ( b ) The contour plot of the mean p i ( r ) as a function of r and t , averaged over all particles that are non-crystalline at t =5,000 s. The particles considered in ( a ) and ( b ) are only those with radii close to the mean radii; see text for details. ( c ) The number of ordered neighbours N o as a function of time for those particles plotted in ( a ) (nucleus particles, solid curve) and ( b ) (non-nucleus particles, dashed curve). Full size image The particles in this experiment are slightly charged and potentially polydisperse in their charge. We therefore note that the effects we see are based on the estimated radius, which likely includes both the core size and the effect of charge: our results show that this estimated radius has a role in nucleation. We cannot disentangle the two effects, but presumably our estimated radius—which relates to how closely particles approach each other—is similar to whatever effective radius is relevant for nucleation. We have developed a general method to estimate the particle sizes in a dense particulate samples where the particle positions are known. This method can be applied to any cases where 3D particle positions can be found; while we have focused on colloidal samples, granular media are quite similar [1] , [44] . We have demonstrated the utility of our method by examining homogeneous colloidal crystal nucleation. While it has been known that nucleation is faster for more monodisperse samples, we find this is true on a quite local scale. Nucleation happens in regions that are locally more monodisperse, and crystal growth proceeds by preferentially incorporating particles close to the mean size. Simulations We simulate four particle suspension systems, which are RCP, colloidal gel, single-component suspension and a binary system. The polydisperse RCP sample is generated using the algorithm of ref. 45 . For the three other cases, we perform 3D Monte Carlo simulations with hard spheres. Additionally for gels, we wish to model colloid-polymer mixtures and so we use the Asakura and Oosawa model [36] . This model leads to a pair interaction between two hard colloidal spheres in a solution of ideal polymers as U ( r )=∞ for r <σ ij , for σ ij ≤ r <σ ij +2 R G , U ( r )=0 for r ≥σ ij +2 R G , where σ ij =( σ i + σ j )/2, σ i is the diameter of particle i , k B is the Boltzmann constant, T is temperature, ρ p is the number density of polymers and R G is the polymer radius of gyration. We fix and where is the mean diameter of the hard spheres. For our single-component and two-component hard-sphere suspensions, particles interact via U ( r )=∞ for r <σ ij , otherwise U ( r )=0. We use 1,024 particles with the mean radius ā =1 and variable polydispersity for all simulations. Experiments The silica particles are fluorescently dyed and are in a refractive index-matched mixture of water and DMSO (dimethyl sulphoxide, (CH 3 ) 2 SO). The silica particles are imaged with a Leica confocal microscope, and their positions are tracked using standard techniques [10] , [35] . For the holographic microscopy of the silica particles, we illuminate the sample with a 445-nm Coherent Cube diode laser mounted above a Nikon Eclipse TE2000-U inverted microscope. The scattered light is collected by a ×1001.4 numerical aperture oil immersion objective (Nikon Plan Apo) and is relayed to a grayscale video camera (NEC TI-324A II) that records at 30 frames per second. Diluted samples are flowed through a glass microfluidic cell and each particle is imaged at least N =10 times. The s.d. of an individual particle's measured radius a from different images is 0.012 μm. The particle's radius is estimated from the average a over the N images that the particle was seen in, and the uncertainty of that estimation is the s.d. divided by . The resulting uncertainty of the particle radius for an individual particle, for N ≥10, is Δ a / a ≲ 0.005. The poly(methyl methacrylate) (PMMA) data come from a prior experiment [11] . This experiment used sterically stabilized PMMA particles that were imaged with a VisiTech confocal microscope and tracked using standard methods [10] , [35] . Each data set has more than 2,800 particles. A more detailed experimental discussion is in ref. 11 . The volume fraction numbers reported in our paper are given to two or three significant digits. The volume fractions are measured by direct counting of particles in a given volume [21] , and converting from the measured number density n to volume fraction φ using φ = nv P using the particle volume vP =(4/3)π a 3 . The particle radii were determined by holographic microscopy (for the silica particles) or by measuring the hydrodynamic radii from dilute suspensions (for the prior PMMA data). The uncertainty of φ with these methods is about 5%, that is, a number such as φ =0.40 is uncertain by about 0.40×0.05=±0.02 (ref. 21 ). Note that this uncertainty is systematic, so for example the data Fig. 4d are correct relative to each other to within the third decimal place, but overall have a systematic uncertainty of ±5%. For example, they may all be 5% larger than the reported values. The same is true for the data of Fig. 4c , which come from different experiments and so have a different systematic error from those of Fig. 4d . Order parameters for crystalline particles We use previously developed order parameters to look for crystalline particles and ordered structure [13] , [43] , [46] . For each particle i , we find its nearest neighbours j and identify unit vectors r̂ ij pointing to the neighbours. We then define a complex order parameter q̂ lm using where c i is the number of nearest neighbours of particle i and Y lm is a spherical harmonic function; we normalize this as where N is a normalization factor such (ref. 13 ). We use l =6. For each particle pair, we compute the complex inner product . Two neighbouring particles are termed 'ordered neighbors' if d 6 exceeds a threshold value of 0.5. For each particle, we focus on N o , the number of ordered neighbours it has at a given time. N o i measures the amount of similarity of structure around neighbouring particles. N o i =0 corresponds to random structure around particle i , while a large value of N o i means that particle i and its neighbour particles have similar surroundings [43] . How to cite this article: Kurita R. et al . Measuring the size of individual particles from three-dimensional imaging experiments. Nat. Commun. 3:1127 doi: 10.1038/ncomms2114 (2012).